Sox17 is indispensable for acquisition and maintenance of arterial identity The functional diversity of the arterial and venous endothelia is regulated through a complex system of signalling pathways and downstream transcription factors. Here we report that the transcription factor Sox17, which is known as a regulator of endoderm and hemopoietic differentiation, is selectively expressed in arteries, and not in veins, in the mouse embryo and in mouse postnatal retina and adult. Endothelial cell-specific inactivation of Sox17 in the mouse embryo is accompanied by a lack of arterial differentiation and vascular remodelling that results in embryo death in utero . In mouse postnatal retina, abrogation of Sox17 expression in endothelial cells leads to strong vascular hypersprouting, loss of arterial identity and large arteriovenous malformations. Mechanistically, Sox17 acts upstream of the Notch system and downstream of the canonical Wnt system. These data introduce Sox17 as a component of the complex signalling network that orchestrates arterial/venous specification. It has long been thought that the different functional and morphological characteristics of arteries and veins are due to their exposure to different hemodynamic conditions, such as shear rate, pressure and flow. However, more recent studies have demonstrated that during embryo development, endothelial cells from arteries and veins have distinct identities even before the establishment of the circulatory system. This suggests that at least in the early stages of endothelial differentiation, genetic determinants have important roles in dictating the arterial/venous fate of endothelial cells [1] , [2] , [3] , [4] . Different signalling pathways and transcription factors have been identified as important players in arterial/venous specification in endothelial cells. These include: the Notch and vascular endothelial growth factor (VEGF) signalling pathways; morphogens, such as Hedgehog and Wnt; the ephrin/Eph systems; and transcription factors, such as COUP-TFII for venous determination, and Foxc1 and Foxc2 for arterial determination [3] , [4] , [5] , [6] , [7] , [8] , [9] , [10] . These pathways can act to promote arterial fate at the expense of venous fate and vice versa . However, reciprocal activation or inhibition between these different signalling systems and the details of how these pathways work together with other, as yet known, factors have not been clarified fully yet. The Notch/Delta-like 4 pathway has been studied extensively in terms of its induction of arterial fate in endothelial cells of the mouse embryo and newborn [9] , [11] , [12] , [13] , [14] . Loss-of-function mutations of the members of the Notch signalling pathway prevent correct arterial differentiation [15] , [16] , [17] . Venous specification is strongly affected in genetically modified mouse embryos that express a gain-of-function mutation of β-catenin, the effector of canonical Wnt signalling. In this model, veins upregulate arterial markers, and by fusing with arteries, form arterio-venous malformations [18] . This phenotype is due to β-catenin-induced Notch signalling, through the transcriptional increase of Dll4 in veins. The Sox (SRY related-HMG box) family of transcription factors has 20 members that have been evolutionarily conserved and that participate in the differentiation of tissues and organs during embryo development [19] , [20] . Sox transcription factors are closely related to the TCF proteins, although they are also DNA-binding HMG-domain proteins. Several members of the Sox family can form complexes with β-catenin and act as transcriptional repressors, and in a few cases, as activators of canonical Wnt transcriptional activity. In some contexts, canonical Wnt/β-catenin signalling can also regulate Sox expression [21] . The SoxF subgroup (Sox7, 17, 18) has an important role in the differentiation of different cell types, including visceral and definitive endoderm and hematopoietic cells [19] , [22] . Furthermore, the SoxF subgroup is necessary for correct cardiovascular development. These three genes are expressed in endothelial cells during development, although only Sox18 is present in the early stages of differentiation of the lymphatic endothelium. Sox18 induces transcription of Prox1, and in this way, it induces the very early stages of lymphatic differentiation [23] . Earlier studies have underlined the redundant roles of the members of the SoxF group in the modulation and development of the cardiovascular system. The compound heterozygosity of Sox17 and Sox18 causes problems in early heart and vascular development in the mouse embryo [24] . The simultaneous loss of Sox7 and Sox18 in Zebra fish alters the arterial/venous differentiation of endothelial cells [25] , [26] , [27] . In human, Sox18 mutations have been associated to a rare pathology known as hypotrichosis–lymphedema–telangiectasia syndrome, which is characterized by altered development of the lymphatic system [28] , [29] . Taken together, these observations support the concept that the SoxF group takes part in vascular remodelling. However, how these transcription factors act and what interactions they have with other signalling pathways are still largely unknown. Here we report that Sox17 is selectively expressed in arterial endothelial cells at the early stages of embryo development, and it maintains the same distribution postnatally and in the adult. Endothelial-cell-specific inactivation of Sox17 in the mouse embryo is accompanied by a lack of arterial differentiation and vascular remodelling, which induces early lethality in utero . In the postnatal retina vasculature, abrogation of Sox17 expression in endothelial cells leads to vascular hypersprouting and large arterio-venous malformations. Large and medium size arteries lose their identity and acquire venous markers instead. In the search for a possible connection between Sox17 and the other transcription systems, we found that Sox17 acts upstream of the Notch system and downstream of the canonical Wnt system. These data introduce Sox17 as a novel factor in the complex signalling network that orchestrates arterial/venous differentiation, whereby Sox17 acts as a link between the canonical Wnt and Notch signalling systems. Sox17 is expressed in embryonic and adult arteries By immunostaining, selective nuclear-associated expression of Sox17 was seen in the arterial endothelium both in the embryo itself and in the yolk sac ( Fig. 1a,b ). The cells positive for Sox17 also expressed ephrinB2, a recognized marker of arterial differentiation ( Fig. 1a,b , Supplementary Fig. S1A ). 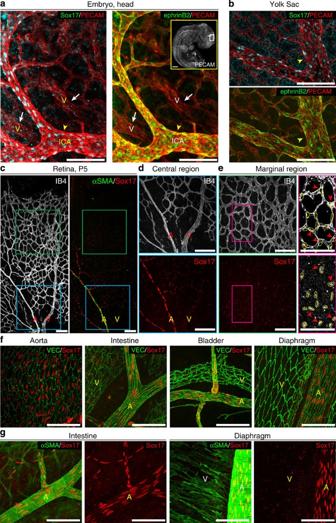Figure 1: Selective expression of Sox17 in developing and mature arteries. (a,b) Confocal analysis of whole-mountephrinB2/β-gal reporter mice. The vasculature of E10.5 embryo head (a) and yolk sac (b) was stained with PECAM (red),ephrinB2/β-gal (green) and Sox17 (light blue). Nuclear staining of Sox17 is seen in the internal carotid artery (ICA, yellow arrowhead), which also expressedephrinB2, while the veins (V, white arrows) are negative. Inset: PECAM staining of the whole embryo showing the area of the head that was analysed. (b) Sox17 expression (light blue) in the E10.5 yolk sac is restricted to large arteries (yellow arrowhead), which also expressedephrinB2.(c–e) Analysis of the vasculature in whole-mount retina. P5, retina from control was stained with isolectin B4 (IB4, white), αSMA (green) and Sox17 (red). Sox17 is highly expressed in large and small arteries (A) while veins (V) are almost negative. Higher magnifications of the central (d) and marginal (e) areas of the retina are shown. Binarized images of Sox17 and isolectin B4 from boxed area in panel (e) were obtained by imposing a threshold of 40 and 78 a.u., respectively. Sox17-positive nuclei are highlighted in yellow and indicated by arrowheads (seeSupplementary Fig. S1Bfor quantification). (f,g) Artery-specific Sox17 staining (red) of the adult mouse vasculature. VE-cadherin antibody (VEC, green) stained both arteries (A) and veins (V) in the different tissues and organs (as indicated). Sox17 was detected only in the arteries. In the intestine and diaphragm, the arteries were labelled by αSMA staining (green) (g). Scale bar, 100 μm. Figure 1: Selective expression of Sox17 in developing and mature arteries. ( a , b ) Confocal analysis of whole-mount ephrinB2 /β-gal reporter mice. The vasculature of E10.5 embryo head ( a ) and yolk sac ( b ) was stained with PECAM (red), ephrinB2/ β-gal (green) and Sox17 (light blue). Nuclear staining of Sox17 is seen in the internal carotid artery (ICA, yellow arrowhead), which also expressed ephrinB2 , while the veins (V, white arrows) are negative. Inset: PECAM staining of the whole embryo showing the area of the head that was analysed. ( b ) Sox17 expression (light blue) in the E10.5 yolk sac is restricted to large arteries (yellow arrowhead), which also expressed ephrinB2. ( c – e ) Analysis of the vasculature in whole-mount retina. P5, retina from control was stained with isolectin B4 (IB4, white), αSMA (green) and Sox17 (red). Sox17 is highly expressed in large and small arteries (A) while veins (V) are almost negative. Higher magnifications of the central ( d ) and marginal ( e ) areas of the retina are shown. Binarized images of Sox17 and isolectin B4 from boxed area in panel ( e ) were obtained by imposing a threshold of 40 and 78 a.u., respectively. Sox17-positive nuclei are highlighted in yellow and indicated by arrowheads (see Supplementary Fig. S1B for quantification). ( f , g ) Artery-specific Sox17 staining (red) of the adult mouse vasculature. VE-cadherin antibody (VEC, green) stained both arteries (A) and veins (V) in the different tissues and organs (as indicated). Sox17 was detected only in the arteries. In the intestine and diaphragm, the arteries were labelled by αSMA staining (green) ( g ). Scale bar, 100 μm. Full size image In the retina of newborn mice at P5, Sox17 was highly expressed in large and small arteries ( Fig. 1c,d ), while Sox17 expression was very weak, and barely detectable, in veins and small capillaries ( Fig. 1d ). In the marginal area of the retina, where blood vessels were actively growing, there was only a relatively weak staining of Sox17 ( Fig. 1e , see endothelial cell nuclei within the dotted lines). The average fluorescence signal intensity of the nuclei was 200 (±30) arbitrary units (a.u.) in the artery endothelial cells, and 50 (±10) a.u. in the veins and capillaries (per 100 nuclei in each group; Supplementary Fig. S1B ). In the adult, Sox17 was strongly expressed in arterial endothelial cells, but was absent or weakly expressed in veins, which suggests that sustained activation of this transcription factor might contribute to the maintenance of arterial identity also after vascular maturation ( Fig. 1f,g ). Higher expression of Sox17 was also detected in cultured human aortic endothelial cells as compared with umbilical vein endothelial cells ( Supplementary Fig. S1C ) and in freshly isolated mesenteric arteries as compared with veins ( Supplementary Fig. S1D ). Sox17 is required for vascular growth and arterial differentiation We then investigated whether Sox17 is required for correct vascular development and for arterial endothelial cell specification. To this end, we first crossed Sox17 flox/flox mice with Tie2 -Cre mice to produce Sox17 ECKO mice. Inactivation of Sox17 induced in utero lethality in 100% of the embryos, within the E10.5 and E12.5 developmental stages. As shown in Supplementary Fig. S1E,F , these Sox17 ECKO mice embryos showed major alterations in vascular remodelling and the development of large arteries was largely absent in all of the organs examined. The intersomitic vessels showed defective patterning, and the vasculature in the yolk sac failed to undergo remodelling, thus missing the correct arterial/venous differentiation (see Supplementary Fig. S1E for the yolk sac, and Supplementary Fig. S1F for the head vasculature and the intersomitic vessels). These data are consistent with previously shown vascular alterations in Sox17 null embryos [22] . To investigate the role of Sox17 in vascular development at the postnatal stages, we crossed the Sox17 flox/flox mice with Cdh5(PAC)- Cre-ER T2 mice [30] , to produce Sox17 iECKO mice and we induced recombination by tamoxifen injection at the P1 postnatal stage. At P5, the endothelial cells of the Sox17-deficient vessels showed a small, but non-significant, increase in the number of tip cells in the vascular growing area at the periphery of the retina ( Fig. 2a,b ; quantification in Fig. 2c,d ). This was further enhanced at P9 ( Fig. 2b ), and up to P12 (quantification in Fig. 2d ). In addition, the growing front of the retina of these Sox17 iECKO mice showed a higher vascular density due to the active, multidirectional hypersprouting of the vasculature ( Fig. 2a–d ). The advancing of the vasculature across the vitreal surface was also slightly, and significantly, reduced at P9 ( Fig. 2b ; quantification in Fig. 2c,d ). Through a closer analysis of the sprouting vessels we observed that the endothelial cells at the stalk of Sox17 iECKO mice ( Fig. 2e , right panels and Supplementary Fig. S2C ) maintained a highly dynamic formation of filopodia like if they did not receive the inhibitory Notch signal by the tip cells. The remarkable multidirectional hypersprouting of the vessels at the periphery of the retina vasculature in these Sox17 iECKO mice is shown at higher magnification in Fig. 2f , right panels and in Supplementary Movie 1 (see also Supplementary Fig. S2A for lower magnification). As sprouting tip cells are in multiple layers the overall staining of Dll4 appears more intense (see Fig. 2g ). 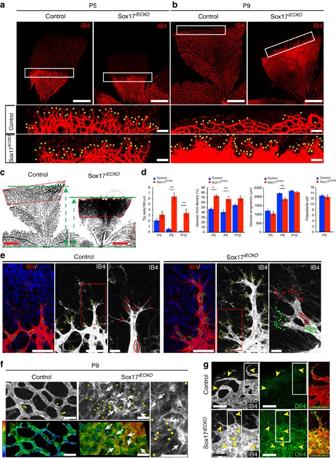Figure 2: Deletion of Sox17 alters vascular development. (a,b) Isolectin B4 (IB4) staining of P5, and P9 retinas from control andSox17iECKOnewborn mice shows marked defects in vascular development. Higher magnification of the angiogenic front (boxed areas) are shown and tip cells are indicated by yellow dots. (c,d) Quantification of vascular parameters in retinas from control andSox17iECKOmice. Binarized images of retinas (P9) from control andSox17iECKO(c, left and right, respectively), as an examples of the quantification performed in (d). The vascular front density was measured in the areas highlighted in red, while vascular progression was measured as the average distance covered by the growing vessels (see green arrows inc). The quantification of the tip cells per length, the vascular front density, the vascular progression and the number of filopodia per tip cell are shown in (d). Retinas from control andSox17iECKO(blue and red columns, respectively) at P5, P9 and P12 are shown. Data are means ±s.d. of at least five mice per group. (e) Detailed analysis of vascular sprouts stained with Isolectin B4 in control andSox17iECKOretinas. Tip cells nuclei are highlighted by yellow circles (see alsoSupplementary Fig. S2Cand Methods for details) and filopodia protrusions by yellow dots (middle panels). Higher magnification of red boxed areas are shown on the right panels where tip cells nuclei and corresponding filopodia are colours coded. (f) High magnification of the angiogenic front show multidirectional hyper sprouting in theSox17iECKOvasculature. Tip cells growing above the vascular plane are indicated by arrows; filopodia are also indicated as yellow dots. Bottom panels show depth-coded stacks (see Methods for details). Tip cells indicated by arrows are located above vascular plexus (green). (g) Higher magnification of Isolectin B4 (IB4, white) and Dll4 (green) staining at the vascular front shows high expression of Dll4 inSox17iECKOhyper sprouting retinas (lower panels, yellow arrowheads). Control tip cells are shown in the upper panel. Scale bar, 500 μm (top panelsa–c); Scale bar, 100 μm (bottom panelsa,b,e); Scale bar, 25 μm (magnifications ofe–g). *P<0.05; **P<0.01, two-tailedt-test assuming unequal variances. Figure 2: Deletion of Sox17 alters vascular development. ( a , b ) Isolectin B4 (IB4) staining of P5, and P9 retinas from control and Sox17 iECKO newborn mice shows marked defects in vascular development. Higher magnification of the angiogenic front (boxed areas) are shown and tip cells are indicated by yellow dots. ( c , d ) Quantification of vascular parameters in retinas from control and Sox17 iECKO mice. Binarized images of retinas (P9) from control and Sox17 iECKO ( c , left and right, respectively), as an examples of the quantification performed in ( d ). The vascular front density was measured in the areas highlighted in red, while vascular progression was measured as the average distance covered by the growing vessels (see green arrows in c ). The quantification of the tip cells per length, the vascular front density, the vascular progression and the number of filopodia per tip cell are shown in ( d ). Retinas from control and Sox17 iECKO (blue and red columns, respectively) at P5, P9 and P12 are shown. Data are means ±s.d. of at least five mice per group. ( e ) Detailed analysis of vascular sprouts stained with Isolectin B4 in control and Sox17 iECKO retinas. Tip cells nuclei are highlighted by yellow circles (see also Supplementary Fig. S2C and Methods for details) and filopodia protrusions by yellow dots (middle panels). Higher magnification of red boxed areas are shown on the right panels where tip cells nuclei and corresponding filopodia are colours coded. ( f ) High magnification of the angiogenic front show multidirectional hyper sprouting in the Sox17 iECKO vasculature. Tip cells growing above the vascular plane are indicated by arrows; filopodia are also indicated as yellow dots. Bottom panels show depth-coded stacks (see Methods for details). Tip cells indicated by arrows are located above vascular plexus (green). ( g ) Higher magnification of Isolectin B4 (IB4, white) and Dll4 (green) staining at the vascular front shows high expression of Dll4 in Sox17 iECKO hyper sprouting retinas (lower panels, yellow arrowheads). Control tip cells are shown in the upper panel. Scale bar, 500 μm (top panels a – c ); Scale bar, 100 μm (bottom panels a , b , e ); Scale bar, 25 μm (magnifications of e – g ). * P <0.05; ** P <0.01, two-tailed t -test assuming unequal variances. Full size image The arterial/venous differentiation appeared altered in the absence of Sox17. In these Sox17 iECKO pups, in the absence of Sox17 the arteries acquired the expression of endomucin, a selective marker of large veins ( Fig. 3a,b compare upper with lower panels; quantification Fig. 3f ) and upregulated Eph4 ( Fig. 3c ). Conversely, Jag1 and Dll4 were significantly reduced ( Fig. 3d,e ). RT–PCR analysis of freshly isolated endothelial cells from the mutant mice (Fig. 6a and Fig. 3g , red columns) also showed that other arterial markers such as Dll4, Notch4 and CXCR4 were reduced and venous markers as COUP-TFII was increased. 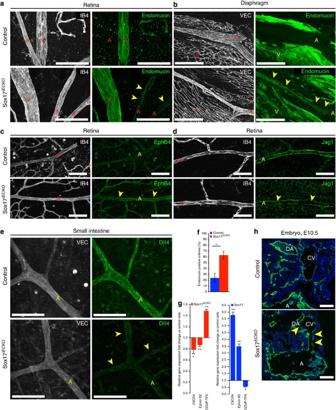Figure 3: Altered arterial and venous differentiation in the absence of Sox17. Analysis of the vasculature of retina, diaphragm and small intestine at P9. (a) Whole-mount immunofluorescence for Isolectin B4 (IB4, white) and endomucin (green) of control andSox17iECKOretinas. Endomucin is expressed in control veins (V). Arrowheads indicate endomucin-positive arteries (A) inSox17iECKOmouse. (b) Staining for VE-cadherin (VEC, white) and endomucin (green) of vessels of control andSox17iECKOmice diaphragm. Arrowheads indicate an artery endomucin positive inSox17iECKOmouse. Quantification of data in (a,b) is shown in panelf(see below). (c) Immunostaining for Isolectin B4 (IB4, white) and EphB4 (green) of control andSox17iECKOretinas. The arrowheads indicate the EphB4 staining in the arteries ofSox17iECKOmouse. (d) Isolectin B4 (IB4, white) and Jag1 (green) staining of the retina vasculature in control and Sox17iECKOmice. The arrowheads point to decreased Jag1 staining inSox17iECKOmouse. (e) Immunofluorescence for VE-cadherin (VEC, white) and Dll4 (green) staining in the vasculature of the intestine in control andSox17iECKOmice. Arterial Dll4 staining is strongly reduced (see arrowheads) inSox17iECKOmice. (f) Quantification of endomucin-positive arteries in control (blue) andSox17iECKO(red) retinas. Data are expressed as percentages of total vessels ±s.d. (n>20). (g) qRT–PCR analysis of control andSox17iECKOlungs derived endothelial cells (red columns) and cultured venous endothelial cells infected with Sox17 (blue columns). Modifications induced in the expression of arterial (CXCR4, ephrinB2) and venous markers (COUP-TFII) are reported. The RNA level obtained for control was set to 1 and the ratio forSox17iECKOversus control or venous endothelial cells infected with Sox17 versus control is shown for each gene. Standard deviation of control values did not exceed 10% of the means. Scale bar, 100 μm; **P<0.01; *P<0.05, two-tailedt-test assuming unequal variances. (h) Confocal analysis of cryosections stained with PECAM (green) and DAPI (blue) of control andSox17ECKOembryos (E10.5) revealed the presence of arteriovenous shunts (arrowheads) leading to a bypass circulation. Scale bar, 200 μm. Figure 3: Altered arterial and venous differentiation in the absence of Sox17. Analysis of the vasculature of retina, diaphragm and small intestine at P9. ( a ) Whole-mount immunofluorescence for Isolectin B4 (IB4, white) and endomucin (green) of control and Sox17 iECKO retinas. Endomucin is expressed in control veins (V). Arrowheads indicate endomucin-positive arteries (A) in Sox17 iECKO mouse. ( b ) Staining for VE-cadherin (VEC, white) and endomucin (green) of vessels of control and Sox17 iECKO mice diaphragm. Arrowheads indicate an artery endomucin positive in Sox17 iECKO mouse. Quantification of data in ( a , b ) is shown in panel f (see below). ( c ) Immunostaining for Isolectin B4 (IB4, white) and EphB4 (green) of control and Sox17 iECKO retinas. The arrowheads indicate the EphB4 staining in the arteries of Sox17 iECKO mouse. ( d ) Isolectin B4 (IB4, white) and Jag1 (green) staining of the retina vasculature in control and Sox17 iECKO mice. The arrowheads point to decreased Jag1 staining in Sox17 iECKO mouse. ( e ) Immunofluorescence for VE-cadherin (VEC, white) and Dll4 (green) staining in the vasculature of the intestine in control and Sox17 iECKO mice. Arterial Dll4 staining is strongly reduced (see arrowheads) in Sox17 iECKO mice. ( f ) Quantification of endomucin-positive arteries in control (blue) and Sox17 iECKO (red) retinas. Data are expressed as percentages of total vessels ±s.d. ( n >20). ( g ) qRT–PCR analysis of control and Sox17 iECKO lungs derived endothelial cells (red columns) and cultured venous endothelial cells infected with Sox17 (blue columns). Modifications induced in the expression of arterial (CXCR4, ephrinB2) and venous markers (COUP-TFII) are reported. The RNA level obtained for control was set to 1 and the ratio for Sox17 iECKO versus control or venous endothelial cells infected with Sox17 versus control is shown for each gene. Standard deviation of control values did not exceed 10% of the means. Scale bar, 100 μm; ** P <0.01; * P <0.05, two-tailed t -test assuming unequal variances. ( h ) Confocal analysis of cryosections stained with PECAM (green) and DAPI (blue) of control and Sox17 ECKO embryos (E10.5) revealed the presence of arteriovenous shunts (arrowheads) leading to a bypass circulation. Scale bar, 200 μm. Full size image Furthermore, detailed analysis of cryosections of Sox17 ECKO embryos at E10.5 showed fusion between the cardinal vein and the dorsal aorta (DA) ( Fig. 3h ) leading to the formation of a bypass circulation from the DA to the sinus venosus region of the heart. The presence of this type of shunts is typical of conditions were arterial–venous identity is lost [14] . The arterial coverage with αSMA, NG2 and Desmin-positive cells was significantly reduced and/or altered in these arteries ( Fig. 4a,d ). The lumen of the veins was frequently enlarged ( Fig. 4a , lower panel) and vascular lacunae were seen at the venous front ( Supplementary Fig. S2B , compare upper with lower panels). 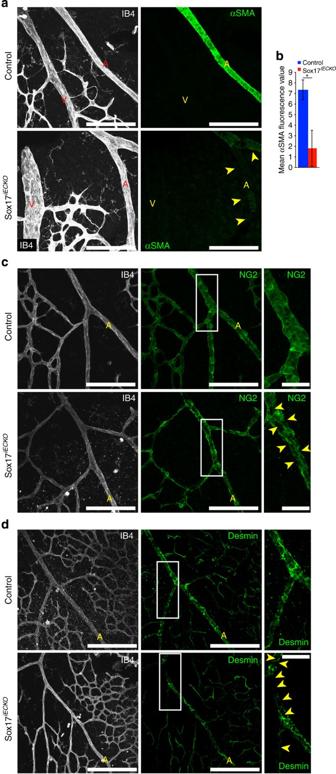Figure 4: Impairment of mural cells coverage in the absence of Sox17. (a–d) Analysis of the control andSox17iECKOretinal vasculature by whole-mount staining for Isolectin B4, αSMA, NG2 and Desmin. (a,b) Isolectin B4 (IB4, white) and αSMA (green) staining. Arrowheads indicate αSMA-negative arteries inSox17iECKOmice. Quantification of αSMA fluorescence intensity in arteries of control andSox17iECKO(blue and red, respectively) is shown in (b). Data are expressed as mean fluorescence ±s.d. (n>3 mice per group) *P<0.01, two-tailedt-test assuming unequal variances. (c) Isolectin B4 (IB4, white) and NG2 (green) staining. (d) Isolectin B4 (IB4, white) and Desmin (green) staining. Higher magnification of the insets is shown in the right panels. Arrowheads indicate regions of incomplete pericyte coverage inSox17iECKOmice. These cells appear poorly organized around the vessel wall leaving relatively large, uncovered areas. Scale bar, 25 μm in magnifications and 100 μm elsewhere. Figure 4: Impairment of mural cells coverage in the absence of Sox17. ( a – d ) Analysis of the control and Sox17 iECKO retinal vasculature by whole-mount staining for Isolectin B4, αSMA, NG2 and Desmin. ( a , b ) Isolectin B4 (IB4, white) and αSMA (green) staining. Arrowheads indicate αSMA-negative arteries in Sox17 iECKO mice. Quantification of αSMA fluorescence intensity in arteries of control and Sox17 iECKO (blue and red, respectively) is shown in ( b ). Data are expressed as mean fluorescence ±s.d. ( n >3 mice per group) * P <0.01, two-tailed t -test assuming unequal variances. ( c ) Isolectin B4 (IB4, white) and NG2 (green) staining. ( d ) Isolectin B4 (IB4, white) and Desmin (green) staining. Higher magnification of the insets is shown in the right panels. Arrowheads indicate regions of incomplete pericyte coverage in Sox17 iECKO mice. These cells appear poorly organized around the vessel wall leaving relatively large, uncovered areas. Scale bar, 25 μm in magnifications and 100 μm elsewhere. Full size image Sox17 is upstream of Notch signalling The observed phenotype of these Sox17 ECKO embryos and of the Sox17 iECKO retina vasculature was very close to that of the embryos and retina vasculature of Notch-signalling-deficient mice [15] , [16] , [17] . It was therefore important to understand the relationships between Notch and Sox17 signalling in arterial specification. We first tested the possibility that Notch is upstream of Sox17 expression. Treatment of newborn mice with the Notch signalling inhibitor N -[ N -(3,5-difluorophenacetyl)-L-alanyl]- S -phenylglycine t -butyl ester (DAPT) did not change the Sox17 expression of freshly isolated lung endothelial cells ( Fig. 5a ), while, as expected, DAPT inhibited the expression of the Notch-dependent transcription factors Hes, Hey1 and Hey2. DAPT treatment of the pups did not modify Sox17 expression in the vessels of the retina ( Fig. 5b ) confirming the RT–PCR data obtained from freshly isolated endothelial cells from DAPT-treated pups ( Fig. 5a ). Sox17 expression was also not changed in Rbpj iECKO pups retina ( Fig. 5c ) and mRNA extracts from lungs ( Fig. 5d ). In both model systems, the Notch target genes where, instead, downregulated as expected ( Fig. 5a,e ). Consistently, also in Dll4 iECKO ( Fig. 5f ) Sox17 staining remained unchanged. 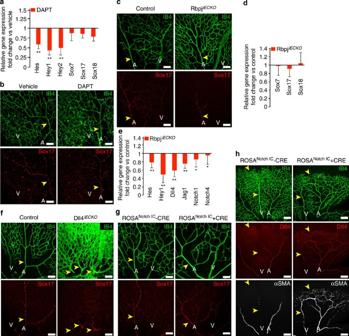Figure 5: Sox17 is upstream of Notch signalling. (a) qRT–PCR analysis of freshly isolated endothelial cells from lungs of vehicle or DAPT-treated pups (P6). DAPT does not affect the expression of Sox17, while inhibits the expression of Hes, Hey1 and Hey2. Data are expressed as fold change versus vehicle and are means ±s.d. from cells obtained from at least four mice per group. The s.d. of the values obtained in vehicle-treated mice did not exceed 10% of the mean. (b) Retina whole-mount immunostaining for Isolectin B4 (IB4, green) and Sox17 (red) after vehicle (left) or DAPT (right) treated pups (P6). Inhibition of Notch signalling does not significantly change Sox17 expression (arrowheads). (c) Whole-mount immunofluorescence for Isolectin B4 (IB4, green), and Sox17 (red) of P6 control andRbpjiECKOretinas. The genetic ablation of Rbpj does not change the expression of Sox17 (arrowheads). (d,e) qRT–PCR analysis ofRbpjiECKOP6 mouse lungs. The genetic ablation of Rbpj does not change the expression of Sox17 (d), while it inhibits the expression of Hes, Hey1, Dll4, Jag1, Notch1 and Notch4. Data are expressed as fold change versus controls and are means ±s.d. from at least three mice per group. The s.d. of the values obtained in control animals did not exceed 10% of the mean. (f) Whole-mount immunofluorescence for Isolectin B4 (IB4, green), and Sox17 (red) of P6 control andDll4iECKOretinas. The genetic ablation of Dll4 does not change the expression of Sox17 (right panels, arrowheads). (g) Isolectin B4 (IB4, green) and Sox17 (red) staining of P6 retinas from control (ROSANotch IC-CRE) and the endothelial-cell-specific gain-of-function mutant of Notch signaling (ROSANotch IC+CRE). Activation of Notch signaling does not significantly change Sox17 expression (arrowheads). The upregulation and ectopic expression of αSMA (white) and Dll4 (red) in veins is shown in (h), see arrowheads. Columns are means ±s.d. of triplicates from a representative experiment. *P<0.05; **P<0.01, two-tailedt-test assuming unequal variances. Scale bar, 100 μm. Figure 5: Sox17 is upstream of Notch signalling. ( a ) qRT–PCR analysis of freshly isolated endothelial cells from lungs of vehicle or DAPT-treated pups (P6). DAPT does not affect the expression of Sox17, while inhibits the expression of Hes, Hey1 and Hey2. Data are expressed as fold change versus vehicle and are means ±s.d. from cells obtained from at least four mice per group. The s.d. of the values obtained in vehicle-treated mice did not exceed 10% of the mean. ( b ) Retina whole-mount immunostaining for Isolectin B4 (IB4, green) and Sox17 (red) after vehicle (left) or DAPT (right) treated pups (P6). Inhibition of Notch signalling does not significantly change Sox17 expression (arrowheads). ( c ) Whole-mount immunofluorescence for Isolectin B4 (IB4, green), and Sox17 (red) of P6 control and Rbpj iECKO retinas. The genetic ablation of Rbpj does not change the expression of Sox17 (arrowheads). ( d , e ) qRT–PCR analysis of Rbpj iECKO P6 mouse lungs. The genetic ablation of Rbpj does not change the expression of Sox17 ( d ), while it inhibits the expression of Hes, Hey1, Dll4, Jag1, Notch1 and Notch4. Data are expressed as fold change versus controls and are means ±s.d. from at least three mice per group. The s.d. of the values obtained in control animals did not exceed 10% of the mean. ( f ) Whole-mount immunofluorescence for Isolectin B4 (IB4, green), and Sox17 (red) of P6 control and Dll4 iECKO retinas. The genetic ablation of Dll4 does not change the expression of Sox17 (right panels, arrowheads). ( g ) Isolectin B4 (IB4, green) and Sox17 (red) staining of P6 retinas from control (ROSA Notch IC -CRE) and the endothelial-cell-specific gain-of-function mutant of Notch signaling (ROSA Notch IC +CRE). Activation of Notch signaling does not significantly change Sox17 expression (arrowheads). The upregulation and ectopic expression of αSMA (white) and Dll4 (red) in veins is shown in ( h ), see arrowheads. Columns are means ±s.d. of triplicates from a representative experiment. * P <0.05; ** P <0.01, two-tailed t -test assuming unequal variances. Scale bar, 100 μm. Full size image On the other hand, an endothelial-cell-specific gain-of-function mutation of Notch signalling (ROSA Notch IC ; see Methods) did not significantly change Sox17 expression in the retina ( Fig. 5g , lower panel). The phenotype of these mice has been previously published [31] and we also report here, as a typical marker of the effect of active Notch signalling, the upregulation and ectopic expression of alpha smooth muscle actin and Dll4 in veins ( Fig. 5h ). Taken together, these data do not support the hypothesis that Sox17 acts downstream of Notch signalling. We then tested whether Sox17 can increase Notch signalling. We first isolated and cultured venous endothelial cells defined as CD45 − /PECAM-1 + /CXCR4 − cells (see Methods and (ref. 32 )), which did not show Sox17 expression. These cells presented low expression of arterial markers as compared with arterial endothelial cells (defined as CD45 − /PECAM-1 + /CXCR4 + cells) ( Supplementary Fig. S3B ). We then infected venous endothelial cells with lentiviral vectors coding for Sox17 or with the transcriptionally inactive Sox18 RaOP (RaOP) mutant that can compete with SoxF for DNA binding [23] . As shown in Fig. 6b , there was a strong increase in NICD translocation to the nucleus only in the Sox17-infected cells (quantification in Fig. 6c ). The transcriptional SoxF competitor RaOP alone was inactive, although it inhibited the effects of Sox17 on Notch signalling, supporting the concept of a specific transcriptional effect of Sox17. 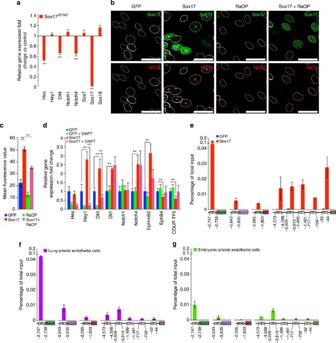Figure 6: Sox17 affects Notch signaling. (a) qRT–PCR analysis of control and Sox17iECKOlungs derived endothelial cells (P6) shows that several members of the Notch signaling pathway (Hes, Dll4 and Notch4) are downregulated by the absence of Sox17. Data are expressed as fold change versus controls and are means ±s.d. from at least three mice per group. The s.d. of the values obtained in control animals did not exceed 10% of the mean. (b) Vein endothelial cells which do not express Sox17 (seeSupplementary Fig. S3A,B) were infected with lentiviral vectors coding for GFP, Sox17, Sox18RaOPor both Sox17 and Sox18RaOPin combination. Immunofluorescence analysis of confluent monolayers stained for Sox17 (green) and NICD (red). Nuclear NICD staining is significantly increased by Sox17 expression (white asterisks), while the Sox18RaOPmutant is inactive. The Sox18RaOPmutant reduced the effects of Sox17 on NICD nuclear staining when it is expressed in combination. Scale bar, 100 μm. Quantification of nuclear fluorescence intensity is reported in (c). Data are means ±s.d. of three experiments. (d) qRT–PCR analysis of Sox17 infected venous endothelial cells (see above). Sox17 expression (red columns) upregulates several members of the Notch signaling pathway, as Hey1, Dll4, Dll1 and Notch4, and arterial markers, such as ephrinB2. Conversely, venous markers, EphB4 and COUP-TFII are downregulated. DAPT treatment (magenta columns) prevent the Sox17-induced upregulation of Hey1 and Dll4. Data are means ±s.d. of four experiments. (e–g) ChIP analysis of Sox17 interaction with the promoters of Notch4, Notch 1, Dll1 and Dll4. The positions of the putative Sox17-binding sites for all the genes analysed are indicated. Chromatin from cultured endothelial cells was immunoprecipitated with Sox17 antibody and qRT–PCR on the indicated regions was carried out. The levels of DNA are normalized to input. (e) ChIP analysis of venous cells infected with GFP (blue) or Sox17 (red); (f) ChIP analysis of arterial cells from lungs expressing endogenous levels of Sox17 (violet); (g) ChIP analysis of arterial cells of embryonic origins expressing endogenous levels of Sox17 (green). Columns are means ±s.d. of triplicates from a representative experiment. *P<0.05; **P<0.01, two-tailedt-test assuming unequal variances. Figure 6: Sox17 affects Notch signaling. ( a ) qRT–PCR analysis of control and Sox17 iECKO lungs derived endothelial cells (P6) shows that several members of the Notch signaling pathway (Hes, Dll4 and Notch4) are downregulated by the absence of Sox17. Data are expressed as fold change versus controls and are means ±s.d. from at least three mice per group. The s.d. of the values obtained in control animals did not exceed 10% of the mean. ( b ) Vein endothelial cells which do not express Sox17 (see Supplementary Fig. S3A,B ) were infected with lentiviral vectors coding for GFP, Sox17, Sox18 RaOP or both Sox17 and Sox18 RaOP in combination. Immunofluorescence analysis of confluent monolayers stained for Sox17 (green) and NICD (red). Nuclear NICD staining is significantly increased by Sox17 expression (white asterisks), while the Sox18 RaOP mutant is inactive. The Sox18 RaOP mutant reduced the effects of Sox17 on NICD nuclear staining when it is expressed in combination. Scale bar, 100 μm. Quantification of nuclear fluorescence intensity is reported in ( c ). Data are means ±s.d. of three experiments. ( d ) qRT–PCR analysis of Sox17 infected venous endothelial cells (see above). Sox17 expression (red columns) upregulates several members of the Notch signaling pathway, as Hey1, Dll4, Dll1 and Notch4, and arterial markers, such as ephrinB2. Conversely, venous markers, EphB4 and COUP-TFII are downregulated. DAPT treatment (magenta columns) prevent the Sox17-induced upregulation of Hey1 and Dll4. Data are means ±s.d. of four experiments. ( e – g ) ChIP analysis of Sox17 interaction with the promoters of Notch4, Notch 1, Dll1 and Dll4. The positions of the putative Sox17-binding sites for all the genes analysed are indicated. Chromatin from cultured endothelial cells was immunoprecipitated with Sox17 antibody and qRT–PCR on the indicated regions was carried out. The levels of DNA are normalized to input. ( e ) ChIP analysis of venous cells infected with GFP (blue) or Sox17 (red); ( f ) ChIP analysis of arterial cells from lungs expressing endogenous levels of Sox17 (violet); ( g ) ChIP analysis of arterial cells of embryonic origins expressing endogenous levels of Sox17 (green). Columns are means ±s.d. of triplicates from a representative experiment. * P <0.05; ** P <0.01, two-tailed t -test assuming unequal variances. Full size image Sox17 infected venous endothelial cells upregulated members of the Notch signalling pathway, including Hey1, Dll4, Dll1 and Notch4, and arterial markers, such as CXCR4 and ephrinB2 ( Fig. 6d , red columns and Fig. 3c blue columns). Conversely, venous markers, EphB4 and COUP-TFII were downregulated ( Fig. 6d , red colums and Fig. 3g , blue columns). To investigate which of these markers were upregulated by Sox17 directly and not indirectly through Notch activation we incubated Sox17 expressing cells with DAPT. As reported in Fig. 6d (magenta columns), with the exception of Hes, Hey 1 and Dll4, which were downregulated by DAPT, Notch4 and Dll1 were upregulated by Sox17 also in the presence of Notch inhibition. To investigate whether Sox17 could interact directly with the promoters of Notch4, Notch1, Dll1 and Dll4 we carried out chromatin immunoprecipitation assay (ChIP). These experiments were performed in venous endothelial cell infected with Sox17 ( Fig. 6e ), in arterial cells from adult lungs and arterial cells from embryo vasculature ( Fig. 6 panel f and g, respectively). In all the three cell lines Sox17 could bind Notch4 promoter at high affinity ( Fig. 6e–g , left panels). Five consensus sequences were identified in the Dll4 promoter region. Sox17 associates to these regions in the venous cells reconstituted with Sox17 ( Fig. 6e , right panel). The binding to Dll4 promoter in the other two cell lines is weaker and occurs mainly in region B ( Fig. 6f,g , right panels). Sox17 binding to Notch1 promoter, even if weak, occurs in venous endothelial cell infected with Sox17 and in arterial cells from adult lungs. Instead, Sox17 binding to Dll1 promoter is negligible ( Fig. 6e–g , middle panels). These data support the idea that Sox17 acts upstream of Notch signalling in its induction of arterial specification of endothelial cells. The action of this transcription factor appears to be quite complex directly interacting with the promoters of different members of the Notch pathway. As VEGF is known to act upstream of the Notch pathway, we then tested whether Sox17 is downstream or upstream of VEGF signalling. As shown in Supplementary Fig. S3C , upregulation of Sox17 did not significantly change the expression of VEGF-A or its receptors, VEGFR-2 and VEGFR-3. On the other hand, VEGF activation of these cells did not increase Sox17 ( Supplementary Fig. S3A ). Canonical Wnt signalling upregulates Sox17 expression In a previous study, we reported that endothelial-specific activation of canonical Wnt signalling prevented correct venous differentiation. In this model, the veins acquired arterial markers and downregulated venous markers [18] . Wnt signalling in the retina and embryo vasculature can induce a strong increase in Sox17 expression [33] . Consistently, Sox17 was markedly increased in freshly isolated endothelial cells from β-catenin gain-of-function mouse embryo and yolk sac ( Fig. 7a,b ). In vivo , in the vasculature of the β-catenin gain-of-function mouse embryo and yolk sac ( Fig. 7c,d ), large vessels were not correctly organized, artery-specific expression of Sox17 was lost and, instead, Sox17 was upregulated in most types of vessels. In the retina of β-catenin loss-of-function pups, Sox17 expression in the small arteries was reduced, while in β-catenin gain-of-function pups was increased ( Fig. 7e ). Importantly, in β-catenin loss-of-function brain vessels (pups, P5) Sox17 expression was essentially abrogated ( Fig. 7f ). 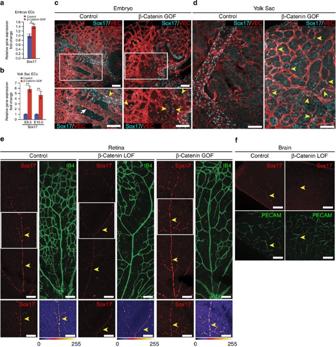Figure 7: Canonical Wnt signaling up-regulates Sox17 expression. (a,b) qRT–PCR analysis of Sox17 expression in endothelial cells derived from β-catenin gain-of-function (GOF) embryos (a) and yolk sac vasculature (b). Data are means ±s.d. of endothelial cells from at least four embryos. (c,d) Whole-mount Sox17 (light blue) and VE-cadherin (VEC, red) staining of E9.5 β-catenin gain-of-function embryos and yolk sacs. The vasculature of the β-catenin gain-of-function mice embryos was severely affected, as reported previously18. Nuclear staining of Sox17 is specifically in arteries of control embryos (c,d; left panels). In contrast, in β-catenin gain-of-function, Sox17 nuclear staining is expressed in most types of vessels (arrowheads). Bottom panels of (c) shows higher magnifications of the boxed areas (white arrow indicates control vein). (e) Confocal images of whole-mount control, β-catenin loss-of-function (LOF) and gain-of-function P6 retinas stained with isolectin B4 (IB4, green) and Sox17 (red). Sox17 expression in the small arteries was reduced in LOF while in GOF pups was increased (see arrowheads). FireLUT (pixels are false coloured according to fluorescent intensity, ranging from dark blue, 0 to white 255) visualization for boxed areas is shown in bottom panels. (f) Confocal images of PECAM (green) and Sox17 (red) stained whole-mounts P5 brains. Sox17 is strongly reduced in β-catenin loss-of-function (LOF). Scale bar, 100 μm. *P<0.05; **P<0.01, two-tailedt-test assuming unequal variances. Figure 7: Canonical Wnt signaling up-regulates Sox17 expression. ( a , b ) qRT–PCR analysis of Sox17 expression in endothelial cells derived from β-catenin gain-of-function (GOF) embryos ( a ) and yolk sac vasculature ( b ). Data are means ±s.d. of endothelial cells from at least four embryos. ( c , d ) Whole-mount Sox17 (light blue) and VE-cadherin (VEC, red) staining of E9.5 β-catenin gain-of-function embryos and yolk sacs. The vasculature of the β-catenin gain-of-function mice embryos was severely affected, as reported previously [18] . Nuclear staining of Sox17 is specifically in arteries of control embryos ( c , d ; left panels). In contrast, in β-catenin gain-of-function, Sox17 nuclear staining is expressed in most types of vessels (arrowheads). Bottom panels of ( c ) shows higher magnifications of the boxed areas (white arrow indicates control vein). ( e ) Confocal images of whole-mount control, β-catenin loss-of-function (LOF) and gain-of-function P6 retinas stained with isolectin B4 (IB4, green) and Sox17 (red). Sox17 expression in the small arteries was reduced in LOF while in GOF pups was increased (see arrowheads). FireLUT (pixels are false coloured according to fluorescent intensity, ranging from dark blue, 0 to white 255) visualization for boxed areas is shown in bottom panels. ( f ) Confocal images of PECAM (green) and Sox17 (red) stained whole-mounts P5 brains. Sox17 is strongly reduced in β-catenin loss-of-function (LOF). Scale bar, 100 μm. * P <0.05; ** P <0.01, two-tailed t -test assuming unequal variances. Full size image In the present study, we show that the Sox17 transcription factor is expressed selectively in small and large arteries in the mouse embryo, postnatal retina and adult. These data are consistent with previous reports that showed that the promoter of Sox17 was predominantly expressed in arterial endothelial cells [34] , [35] , [36] . The high Sox17 expression in arteries of newborn and adult mice reported here supports the idea that this transcription factor is important not only for induction of arterial specification at the early stages of development but also for its maintenance in the mature vasculature. Conditional deletion of Sox17 in endothelial cells of the embryo and postnatal retina indicates that this transcription factor is indispensable for a correct acquisition and maintenance of arterial identity. In a previous study, global deletion of Sox17 did not induce major abnormalities in the embryonic vasculature, including for the DA, intersomitic vessels and microvasculature of different organs [24] . The reasons for this discrepancy probably arise from the mixed genetic background of these mice. As shown in some studies, the members of the SoxF group can act as strain-specific modifiers and can functionally substitute for the inactivation of other members of the group [24] , [37] , [38] . Indeed, mouse Sox17/Sox18 double-null embryos showed severe defects in heart development and anterior DA [24] , [38] . However, as reported in the present study, in a pure C57Bl/6J genetic background, endothelial-specific Sox17 has an important, non-redundant role in endothelial cell growth and arterial specification. The defects that have been described for specific loss of endothelial Sox17 are similar to those described in embryos and newborn mice deficient in Notch signalling [15] , [16] , [17] . Although we were not able to find evidence that inhibition or activation of Notch signalling can influence Sox17 expression, we did see strong activation of Notch signalling by Sox17 expression in different systems. This effect is consistent with the upregulation of elements of the Notch pathway, such as Notch4, Dll4 and Dll1 and the related downstream transcription factors. In agreement with the results reported here, two other reports described, in different systems, an association between the SoxF and the Notch pathway. Clarke et al . [39] showed that Sox17 has a role in the differentiation and expansion of the hemogenic endothelium from ES cells in vitro through the upregulation of Notch1. Sacilotto et al . [36] showed that the arterial-specific upregulation of Dll4 in Zebrafish and the mouse is due to a combinatorial binding of RBPJ/Notch intracellular domain and the SoxF to the gene enhancers of Dll4. Although this work does not specifically refers to Sox17 it is consistent with the observation reported here of a combinatorial effect of Sox17 and Notch in increasing Dll4 expression. In Zebrafish, Sox17 is mostly expressed in the endoderm during gastrulation, and it is not expressed in the vessels. However, simultaneous inactivation of Sox7 and Sox18 by morpholino injection prevents correct arterial/venous specification, with the appearance of arterio–venous shunts. It is likely, therefore, that in the fish the Sox orthologs acquire different activities and specificities [25] , [26] , [27] . An important question is what induces Sox17 upregulation in the vascular system. VEGF is induced by the low oxygen tension, it is present during the development of the retina [40] and can upregulate Dll4 and Notch signalling [1] , [2] , [11] . VEGF is considered to be the major inducer of vascular sprouting and arterial differentiation in this system. In our study, however, we were not able to detect changes in Sox17 expression through VEGF activation of endothelial cells; vice versa , upregulation of Sox17 did not change the expression of VEGFA and its receptors. Yang et al . 35 showed that in tumour-derived endothelial cells, Sox17 increased VEGFR-2 expression. It is possible that the use of different cell types or of a different context, such as the inflammatory tumour stroma, might modify the type of response of the endothelium to this transcription factor. In the present study, we have provided evidence that Sox17 may act downstream of Wnt/β-catenin signalling. We have reported previously that activation of the canonical Wnt pathway upregulates Dll4 and Notch signalling, which, in turn, induce veins to acquire arterial characteristics [18] . Ye et al . [33] reported that Sox17 is a target of Norrin/Frizzled 4 pathway acting through β-catenin signalling in the retina vasculature. In the present study, we have confirmed these data, and shown further that Sox17 is upregulated by β-catenin in both the mouse embryo and yolk sac vasculature. A schematic representation of the interactions among the different signalling pathways in arterial specification is reported in Fig. 8 . 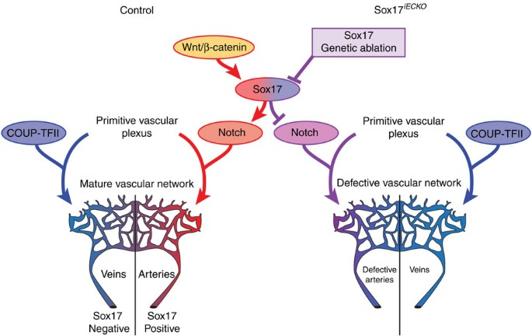Figure 8: Role of Sox 17 on vascular development. Schematic representation of the suggested interaction among the different signaling pathways that regulate arterial/venous specification. Wnt is upstream of Sox17 that, in turn, activates Notch signaling and arterial differentiation. Endothelial-specific inactivation of Sox17 prevents Notch signaling and acquisition of arterial identity by endothelial cells. Figure 8: Role of Sox 17 on vascular development. Schematic representation of the suggested interaction among the different signaling pathways that regulate arterial/venous specification. Wnt is upstream of Sox17 that, in turn, activates Notch signaling and arterial differentiation. Endothelial-specific inactivation of Sox17 prevents Notch signaling and acquisition of arterial identity by endothelial cells. Full size image The direct relevance of the observations reported here in human pathology remains to be clarified. However, reduced β-catenin signalling in the retina is the cause of pathological retinal hypovascularization in Norrie disease [41] . It would be important to understand to what extent reduced Sox17 levels mediated by altered β-catenin signalling influence the development of this disease. Importantly, a multi-stage, genome-wide association study that included a few thousand patients with intracranial aneurism identified a susceptibility locus that contains the Sox17 gene [42] , [43] . The intracranial aneurysms predominated at arterial branch points and sites of shear stress. It is tempting to speculate that altered Sox17 expression can affect arterial differentiation and increase the vascular fragility to hemodynamic stress. Sox17 is upregulated in tumour vasculature, and appears to be involved in angiogenesis and in increasing tumour-cell dissemination [35] . At this stage, we do not know whether and how these effects are related to the observations reported in the present study during physiological vascular development in the embryo and postnatal retina. However, all of these direct and indirect observations underline the crucial role of Sox17 in vascular development and hemostasis. Yang et al . [35] also report that expression of Sox17 induces vascular angiogenesis and abnormalities in Lewis lung carcinoma and, conversely, that Sox17 deletion reduces angiogenesis and causes vascular normalization. It is likely that the role of Sox17 in pathological (tumour vessels) or physiological conditions, as reported here, is different. The paper by Yang et al . [35] shows that Sox17 is strongly increased in LLC tumour vasculature in comparison with normal vessel. However, this is not the case in B16 F10 tumours where the level of Sox17 in the vasculature is much lower. In agreement with this, endothelial deletion of Sox17 leads to changes in vascular proliferation in LLC but not in B16 F10. This underlines that the level of Sox17 is an important determinant for its downstream effects as for other transcription factors (see for instance [44] ). Sox17 high may associate to diverse transcriptional partners inducing different patterns of downstream target genes. In tumours such as LLC the levels of Sox17 in the vasculature are very high and it is not surprising that the downstream effects are not superimposable to those regulated by the physiological concentrations of this transcription factor. Another important variable to consider is the degree of vascular maturation. At late times of tumour (LLC) implantation, abrogation of Sox17 does not cause major effects on the tumour vasculature [35] . For instance, alpha smooth muscle actin-positive pericytes were abundant in vessels of early Sox17 deletion tumours but were reduced in late Sox17 deleted mice (as we observe in the present paper). This suggests that depending on vascular maturation and stability, the response to Sox17 deletion may vary considerably. Genetic experiments and pharmacological inhibition All animal procedures were performed in accordance with the Institutional Animal Care and Use Committee (IACUC), in compliance with the guidelines established in the Principles of Laboratory Animal Care (directive 86/609/EEC) and approved by the Italian Ministry of Health. The following mouse strains were used: Sox17 flox/flox (ref. 22 ), β-catenin flox/flox (ref. 45 ), β-catenin flox(ex3)/flox(ex3) (ref. 46 ), ephrin-B2 (ref. 4 ), Gt(ROSA)26-Sor tm1 (Notch1)Dam/J (ref. 47 ) (a kind gift of Dr D.A. Melton, Harvard University Cambridge, Massachusetts, USA) Cdh5(PAC)- Cre-ER T2 (ref. 30 ), Pdgfb-iCre mice (ref. 48 ), Dll4 flox/flox (ref. 49 ), Rbpj flox/flox (ref. 50 ). For endothelial-cell-specific loss-of-function of Dll4 and Rbpj, mice were interbred with Pdgfb-iCre transgenics [40] , [48] . Endothelial-cell-specific β-catenin loss-of-function and gain-of-function were generated interbreeding β-catenin flox/flox or β-catenin flox(ex3)/flox(ex3) , respectively, with Tie2 -Cre mice or Cdh5(PAC)- Cre-ER T2 (refs 18 , 51 , 52 ). The Sox17 ECKO embryos were generated by mating Sox17 flox/flox mice (a kind gift of Dr S.J. Morrison, Howard Hughes Medical Institute, University of Michigan, Michigan, USA) with Tie2 -Cre mice [51] , to produce the Sox17 flox/+ /Cre + mice. These mice were then interbred with Sox17 flox/flox , to obtain the Sox17 flox/flox /Cre + mice. All of the mouse strains were back-crossed into the C57Bl/6J background. To delete Sox17 in the postnatal vasculature, we interbred Sox17 flox/flox mice with Cdh5(PAC)- Cre-ER T2 mice. Sox17 flox/+ /Cdh5(PAC)- Cre-ER T2+ mice were interbred with Sox17 flox/flox mice to generate litters containing Sox17 flox/flox /Cdh5(PAC)- Cre-ER T2+ ( Sox17 iECKO ) mice and control ( Sox17 flox/flox ) littermates. Cre activity and genetic modifications were induced by subcutaneous injections in the neck skin with 100 μg tamoxifen (Sigma) in every pup of the litter, at P1. Notch signalling was inhibited in the pups by subcutaneous injection with 100 mg kg −1 DAPT (Alexis Bioscience) in 10% ethanol and 90% corn oil or vehicle only, at P4 and P5. The lungs were collected and the endothelial cells isolated at P6, 48 h after the first injection of DAPT. Antibodies The following antibodies were used: anti-VE-cadherin (5 μg ml −1 , BV13, eBioscience), anti-PECAM-1 (1:200, BD), anti-Sox17 (1:200, R&D Systems), anti-αSMA (1:400, FITC-conjugated, Sigma), anti-β-galactosidase (1:500, Abcam), anti-endomucin (1:200, Santa Cruz), anti-Dll4 (1:200, R&D Systems), anti-NICD (1:100, Abcam), anti-EphB4 (1:200, R&D Systems), anti-Jag1 (1:100, Santa Cruz), anti NG2 (1:200, Abcam), anti-desmin (1:200, Abcam) and isolectin-B4 (1:100, Vector Labs). The anti-Sox17 antibody specificity was confirmed by immunostaining of the mice retinas (see Supplementary Fig. S1G ). Alexa Fluor 488, 555 and 647 donkey secondary antibodies were from Invitrogen. Endothelial cell culture and qRT–PCR For the isolation of endothelial cells from embryos, E9.5 to E10.5 embryos were dissected and dissociated with collagenase type I (Roche, 1.5 mg ml −1 ), DNase (Roche, 25 μg ml −1 ) at 37 °C for 1 h and passed through a 40 μm cell stainer [18] . Cells in this flow-through were collected by centrifugation and washed in 0.1% BSA in PBS. The venous endothelial cells were separated with the FACSAria cell-sorting system (BD Biosciences), with the combination of APC-conjugated anti-PECAM-1 (BD), PE-Cy7-conjugated anti-CD45 (eBioscience) and PE-conjugated anti-CXCR4 (eBioscience) [32] antibodies (venous endothelial cells were defined as CD45 − /PECAM-1 + /CXCR4 − ). The endothelial cells were immortalized [52] and lentivirally transduced with Sox17 and Sox18 RaOP cDNAs, subcloned into the lentiviral plasmid pRRLsin.PPTs.hCMV.GFPwpre under the transcription of CMV promoter [23] . DMSO or an equal volume of DAPT (10 μM) dissolved in DMSO was added to the culture cells and incubated for 24 h. Cells were then lysate for RNA extraction. For VEGF stimulation, the endothelial cells were grown to confluence, serum starved (MCDB, 1% BSA) overnight, and then incubated with 80 ng ml −1 VEGF (Peprotech) for 8 h. These cells were then lysed for RNA extraction. Freshly isolated endothelial cells from lungs of Sox17 iECKO (P6) and DAPT-treated mouse pups (see above) were isolated using Dynabeads (Invitrogen) and processed for RNA extraction, as described below [18] . Total RNA from lungs of Rbpj iECKO pups (P6) was isolated as described below [40] . Human endothelial cells isolated from umbilical vein (HUVECs) by treatment with Collagenase (Roche, 0.1%, for 30 min at 37 °C) were routinely cultured [53] ; HAEC were purchased from Life Technologies. Mesenteric arteries and veins were isolated from mice and immediately processed for RNA. All of the types of endothelial cells were grown, in MCDB-131 (GIBCO) with 20% serum. For gene expression analysis, the total RNA was isolated with RNeasy Mini kits (QIAGEN) and 1 μg total RNA was reverse transcribed with random hexamers (High-Capacity cDNA Archive kits; Applied Biosystems) following the manufacturer instructions. Micro fluidic cards (qPCR cards, Applied Biosystems) were created for array profiling of the transcripts of the genes described in Supplementary Table S1 . The cDNAs were amplified using the TaqMan Gene Expression Assay (Applied Biosystems) in an ABI/Prism 7900 HT thermocycler. The relative expression differences represent the means of the results obtained from at least three-independent experiments. ChIP assay ChIP assay was carried out as described [18] , [54] ; briefly, chromatin extracts containing 1 mg of DNA fragments with an average size of 500 bp were immunoprecipitated with 10 μg Sox17 antibody overnight at 4 °C in the presence of protein G magnetic beads (Invitrogen). Bound DNA fragments were eluted and amplified by standard PCR and qRT–PCR with the use of oligonucleotides flanking the assayed promoter regions. Primers used are listed in Supplementary Table S2 . For qRT–PCR analyses, DNA was diluted with specific primers (10 μM each) to a final volume of 25 μl in SYBR green Reaction Mix (Perkin Elmer). Immunofluorescence For cell immunofluorescence, confluent endothelial cells were fixed with 4% paraformaldehyde (PFA) in PBS, followed by permeabilization with 0.5% Triton X-100 for 5 min. The blocking (1 h), primary (2 h) and secondary (1 h) antibodies were in PBS with 2% BSA. The nuclei were visualized using DAPI. Retina immunostaining was carried out with littermates processed simultaneously under the same conditions. To analyse and quantify the retina vascular phenotype, the eyes (P5, P9 and P12) were fixed in 2% PFA for 2 h at 4 °C and dissected. After blocking/permeabilization in 1% BSA, 5% donkey serum and 0.5% Triton-X100 in PBS overnight, the retinas were washed in Pblec Buffer (1% Triton X-100, 1 mM CaCl 2 , 1 mM MgCl 2 and 0.1 mM MnCl 2 in PBS, pH 6.8) and incubated overnight at 4 °C in Pblec buffer containing biotinylated isolectin B4 (IB4) and the primary antibodies. Then the retinas were incubated with fluorophore-conjugated antibodies and with Alexa Fluor 488/555/647 streptavidin (Invitrogen), and mounted with ProLong Gold (Invitrogen). For whole-mount immunostaining [18] , embryos were dissected in PBS and fixed in 4% PFA overnight at 4 °C. After blocking/permeabilization for 3 h in PBS containing 0.3%TX-100 and 5% donkey serum, embryos were incubated overnight at 4 °C with the primary antibodies followed by the species-specific Alexa Fluor-coupled secondary antibodies. Cryostat sections (8–12 μm thick) were cut using a cryotome (Leica), mounted on Superfrost glass slides and dried. Sections were permeabilized for 5 min in PBS containing 0.5% TX-100, blocked in 2% BSA, 5% donkey serum and 0.05% TX-100 in PBS and incubated overnight at 4 °C with the primary antibodies. Secondary detection was performed with Alexa Fluor-coupled secondary antibodies for 3 h at room temperature. Speciments were mounted with Vectashield (Vector Labs). Cerebella (P5) were dissected, fixed and embedded in 3% low melting point agarose and 100 μm sections were cut on vibratome and immunostained. After anaesthesia, mice were perfused for 2 min with fixative (1% PFA in PBS, pH 7.4) from a cannula inserted through the left ventricle into the aorta [55] . The aorta, diaphragm, urinary bladder and intestine were fixed in 1% PFA at pH 7.5 for 1 h, antibodies were diluted in 5% donkey serum in PBS containing 0.3% Triton-X100. The stained tissues were mounted with Vectashield (Vector Labs). Confocal microscopy was performed with Leica TCS SP2 and SP5 confocal microscopes. ImageJ (NIH) was used for the data analysis. The figures were assembled using Adobe Photoshop and Adobe Illustrator. The only adjustments used in the preparation of the figures were for brightness and contrast. For comparison purposes, different sample images of the same antigen were acquired under constant acquisition settings. Image analysis Image analysis was performed using the ImageJ software. Depth-coded stacks were generated using the dedicated plug-in, which assigned a gradient of pseudo-colours that ranging from red to blue (see ‘Depth Index’ in Fig. 2 ), varying according to focal plane depth. The mean fluorescence intensities in Figs 4 , 6 , and Supplementary Fig. S1 were determined as the mean intensities of the fluorescent pixels after segmentation, which was performed by assigning a threshold value (constant within each experiment) of fluorescence for every image. The vessel front density in the retinas was measured as a percentage of pixels with a value greater than the threshold applied for image segmentation. Tip cell nuclei highlighted in Fig. 2e derived from a plane-by-plane analysis of confocal stacks. However, in order to obtain a more comprehensive visualization of the complete sprouts only stack projection are shown. For clarity, an example of a single confocal plane with highlighted nuclei is presented in Supplementary Fig. S2C . Statistical analysis Statistical significance was determined by independent two-tailed t -test assuming unequal variances. How to cite this article: Corada, M. et al . Sox17 is indispensable for acquisition and maintenance of arterial identity. Nat. Commun. 4:2609 doi: 10.1038/ncomms3609 (2013).